Femtosecond X-ray-induced explosion of C60at extreme intensity Understanding molecular femtosecond dynamics under intense X-ray exposure is critical to progress in biomolecular imaging and matter under extreme conditions. Imaging viruses and proteins at an atomic spatial scale and on the time scale of atomic motion requires rigorous, quantitative understanding of dynamical effects of intense X-ray exposure. Here we present an experimental and theoretical study of C 60 molecules interacting with intense X-ray pulses from a free-electron laser, revealing the influence of processes not previously reported. Our work illustrates the successful use of classical mechanics to describe all moving particles in C 60 , an approach that scales well to larger systems, for example, biomolecules. Comparisons of the model with experimental data on C 60 ion fragmentation show excellent agreement under a variety of laser conditions. The results indicate that this modelling is applicable for X-ray interactions with any extended system, even at higher X-ray dose rates expected with future light sources. The recent development of high peak brightness X-ray free-electron lasers [1] (XFELs) has enabled breakthroughs in several fields, including warm dense plasmas [2] and the diffractive imaging of biological macromolecules [3] , [4] , [5] , [6] . The interpretation of these experiments is facilitated by comparison with computational models of the X-ray matter interaction, in which the models are exploring previously untested intensity regimes. Both biomolecule imaging and computational modelling related to molecular structure reconstruction currently attract great interest, receiving recent Nobel Prizes in Chemistry [7] , [8] . Serial femtosecond nanocrystallography [2] , [3] , [4] , [5] and imaging of individual proteins and viruses at atomic resolution call for higher intensity and shorter X-ray pulses [9] , [10] , [11] , [12] , [13] , [14] , [15] , which will allow an image to be acquired before radiation damage destroys the sample. Advances in X-ray focusing capabilities [16] and XFEL peak brightness [17] suggest that a regime of multiple photons absorbed per atom, with dramatic radiation damage occurring within the 10–100 fs X-ray pulse duration, is likely to be reached in the next few years. This regime is essential to achieve the goal of single-particle imaging at the ångstro¨m scale in samples lacking crystal structure to give rise to diffraction peaks. Developing a fundamental understanding of this new regime is therefore vital to progress in X-ray imaging. Our results are also relevant to studies of matter under extreme conditions being investigated by both optical and X-ray lasers wherein data interpretation often relies on atomic and molecular data and models [18] , [19] . Study of C 60 fragmentation dynamics under high femtosecond X-ray flux provides key insight on molecular dynamics in carbon-bonded molecules, to better understand the influence of intra-pulse radiation damage on molecular X-ray imaging. These considerations motivated the present investigation of femtosecond X-ray-induced fragmentation of an intermediate-sized molecule. During the last decade, several models have been developed for studying the time evolution of small and large samples irradiated by XFEL pulses [11] , [20] , [21] , [22] , [23] , [24] , [25] , [26] , [27] , [28] . Under these extreme conditions, the sample was predicted to become highly excited (for example, all atoms can be ionized). Systems relevant for coherent imaging are typically large (100–100,000 atoms) and handling such a problem with fully quantum mechanical methods is numerically not feasible today. All developed models describe the dynamics of atoms/ions and electrons that appear in the continuum after ionizations by classical physics, and contain phenomenological elements alongside parameters derived directly from quantum mechanical calculations. For studies aiming at atomic resolution, theoretical support through molecular dynamics (MD) modelling that provides information about atomic positions is essential. MD modelling has been used to make predictions for bioimaging [11] , [12] , [13] , [14] and has helped to interpret scattering experiments [15] . However, the X-ray scattering measurements central to these studies do not allow access to detailed dynamical information of the individual particles. Therefore, a validation of such a tool based on a direct comparison of dynamical quantities from experiment and modelling is crucial to show that these approaches can make quantitatively correct predictions. Earlier atomic experiments have provided insight on the nature of the interaction of light [29] and heavy [30] atoms with intense X-ray pulses. Here we report important insights for a complex molecule. Specifically, we demonstrate the effects of high per-atom X-ray absorption on the fragmentation dynamics of C 60 molecules in the gas phase. C 60 offers a number of advantages as a benchmark molecule when compared with isolated atoms [29] , [30] , [31] , [32] , [33] , small molecules [34] , [35] , [36] , [37] , [38] , [39] , [40] or van der Waals (vdW) clusters [41] , [42] , from the perspective of radiation damage. C 60 consists of chemically bonded carbon atoms with representative bond lengths and damage processes. Secondary ionization by photo- and Auger electrons, weak in isolated small molecules and absent in atoms, is found to be significant in the dynamics of C 60 under high photon dose rate conditions. Molecular influences on the Auger decay process, which are weak in vdW clusters, are also found to be much stronger in C 60 and must be incorporated in calculations to account for the experimental data. The short C–C bond lengths also lead to far stronger Coulomb repulsion forces between the rapidly charging ions during the X-ray pulse, producing ion–ion forces more representative of chemically bonded systems under high X-ray flux than those seen in vdW clusters. To understand the effects of increased per-atom dose in the photon–molecule interaction, we use the large photoabsorption cross-section of carbon 1s electrons at 485 eV photon energy to reach conditions in which each atom in a C 60 molecule in the X-ray focus absorbs multiple photons during X-ray pulses of 4–90 fs duration. The resulting calibrated model can be scaled to the parameters of a broad variety of experiments, including those typical of biomolecular imaging. Thus, radiation damage dynamics predictions can be made for X-ray interactions at far higher intensity. Femtosecond ionization dynamics The Linac Coherent Light Source (LCLS) XFEL provides femtosecond X-ray pulses of high pulse energy and variable pulse duration. The dominant ionization mechanism in this case is a sequential multiphoton absorption as observed in previous studies of chemically simpler systems, but not yet investigated for a large strongly bonded system like C 60 . Multiple sequential core-level photoionization (P) and subsequent Auger decay (A) events, accompanied by secondary ionization processes, lead to highly charged ionic states of C 60 during the absorption of photons from a single X-ray pulse. As the highly charged parent molecule begins to break up, it and its fragments absorb many photons through several sequential photoionization–Auger (P–A) cycles, leading to highly charged fragment ions. These repeated P–A cycles do not occur in single-photon absorption (for example, in synchrotron light source experiments [43] ). While the experiment helped to identify key processes required for the model, our calculations helped to interpret the data and give detailed insight into the dynamics. For a direct comparison of experiment and theory, the XFEL pulse properties must be known. Calibrations revealed that the XFEL parameters can differ from the nominal values provided by LCLS, for example, the actual pulse duration is 50–60% of the nominal value as also indicated by earlier studies [29] , [34] . Our calibrations indicated that for the nominal pulse durations of 7, 60 and 150 fs full-width at half-maximum recorded with the experimental data, actual pulse durations of 4, 30 and 90 fs, respectively, are more appropriate. We use throughout this article the ‘actual’ calibrated pulse durations, and we refer to these as short (4 fs), intermediate (30 fs) and long pulses (90 fs). The time evolution of C 60 irradiated by a high-intensity XFEL pulse as revealed in detail by modelling is illustrated in Fig. 1 . Early in the X-ray laser pulse, due to photoionization and Auger electron emission, high-energy electrons appear that can escape, leaving behind a highly charged C 60 ion accumulating Coulomb potential energy ( Fig. 1a ). Due to the increasing ion repulsion, C 60 starts to explode, and substantial atomic displacement (~10 Å) occurs within tens of femtoseconds after the first ionization events ( Fig. 1b ). The ionic potential increases and slows down electrons ejected later on during the pulse. Some of the photo- and Auger electrons, together with slow electrons generated via secondary ionizations, are trapped by the increasing ionic potential ( Fig. 1b ). These electrons form a nanoplasma surrounding and penetrating the remnant of the buckyball, while electrons that could escape are already at large distances ( Fig. 1c ). Within the first 100 fs, the fragment ions reach their asymptotic velocity having converted most of the accumulated potential energy into kinetic energy (KE). The electron nanoplasma expands with the carbon ions and a fraction of it evaporates within nanoseconds, while others recombine forming the final detectable ionic charge states ( Fig. 1d ). Although secondary ionization has been previously reported in the case of very large Xe vdW clusters [41] and solid aluminium [19] , our investigation, to the best of our knowledge, reveals for the first time significant collisional ionization within a single molecule exposed to intense X-rays. 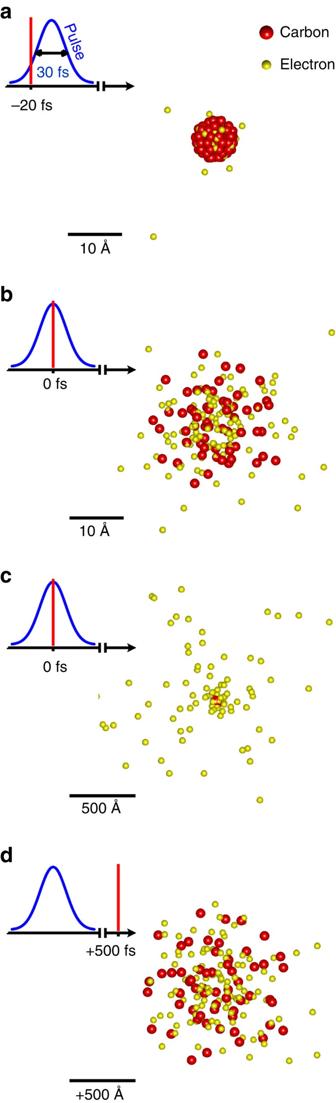Figure 1: Real-space theoretical modelling snapshots of the time evolution of a C60molecule irradiated by an XFEL pulse. The positions of the carbon atoms (red) and electrons (yellow) are shown as a function of time at fine (a,b) and expanded (c,d) spatial scale. The peak intensity of the X-ray pulse occurs att=0. Note that bothbandcshow the system at the same time but on a different spatial scale. Substantial (~10 Å) atomic displacement occurs during the X-ray pulse. At later times, several trapped (quasi-free) electrons remain among the ions, forming a nanoplasma. The pulse duration is 30 fs, with Gaussian pulse shape and a pulse energy of 345 μJ (4.4 × 1012photons with energy 485 eV). The focal spot size is 1.4 × 1.4 μm2. Figure 1: Real-space theoretical modelling snapshots of the time evolution of a C 60 molecule irradiated by an XFEL pulse. The positions of the carbon atoms (red) and electrons (yellow) are shown as a function of time at fine ( a , b ) and expanded ( c , d ) spatial scale. The peak intensity of the X-ray pulse occurs at t =0. Note that both b and c show the system at the same time but on a different spatial scale. Substantial (~10 Å) atomic displacement occurs during the X-ray pulse. At later times, several trapped (quasi-free) electrons remain among the ions, forming a nanoplasma. The pulse duration is 30 fs, with Gaussian pulse shape and a pulse energy of 345 μJ (4.4 × 10 12 photons with energy 485 eV). The focal spot size is 1.4 × 1.4 μm 2 . Full size image Atomic ion yields for C 60 and for atomic carbon At high X-ray fluence, the volume-integrated ion fragment mass spectra are dominated by the atomic ions over the molecular fragments for all of the experimentally realized pulse durations and fluence values. The simulations predict that for fluence above 360 J cm −2 , the molecules fragment completely into atomic ions. Therefore, by selecting the atomic ion fragments, we can focus our study more on the dynamics in the highest fluence region. 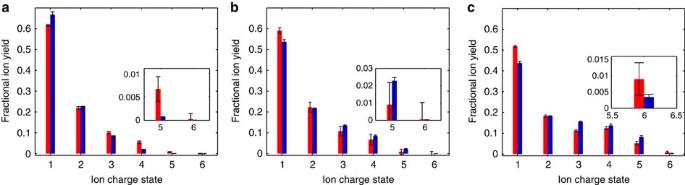Figure 2: Relative carbon ion yield versus charge state. Experimental data (red bars) and calculated results (blue bars) are presented with error estimates (black lines) for experimental data based on Poisson statistics as described in the Methods section. The main error in the calculated data is due to the uncertainty of the pulse parameters, which were determined by assuming ±10% deviation from the nominal pulse energy. Plotted are (a) short pulses, (b) intermediate pulses and (c) long pulses. Insets show higher charge states at magnified vertical scale. Photon energy was 485 eV in all cases. Plots are normalized so that all experimental bars, and all calculation bars, sum to one, respectively. Figure 2 shows measured and modelled atomic C ion yields for short and intermediate pulse durations, at near equal X-ray fluence, and for a long pulse duration at higher fluence. There is very good agreement between the experimental and theoretical results. A common feature of almost all of the charge distributions is that the yield monotonically decreases with increasing charge. For the long pulse, high-fluence case, we observed fully stripped carbon C 6+ . The observation of C 5+ and C 6+ yields has not been previously reported using intense optical lasers [44] , [45] . In the present report, the degree of nonlinearity in sequential multiphoton absorption is extreme—an average of 180 X-ray photons are absorbed per molecule in the X-ray focus, corresponding to 87 keV total energy transfer to the fullerene. This is by far the most nonlinear photoprocess in a molecule ever reported in the X-ray spectrum. Our integrated experimental and theoretical work also demonstrates that electron impact ionization, which plays a key role in matter in extreme conditions’ experiments [18] , [19] , is significant in a molecule containing just 60 atoms. Figure 2: Relative carbon ion yield versus charge state. Experimental data (red bars) and calculated results (blue bars) are presented with error estimates (black lines) for experimental data based on Poisson statistics as described in the Methods section. The main error in the calculated data is due to the uncertainty of the pulse parameters, which were determined by assuming ±10% deviation from the nominal pulse energy. Plotted are ( a ) short pulses, ( b ) intermediate pulses and ( c ) long pulses. Insets show higher charge states at magnified vertical scale. Photon energy was 485 eV in all cases. Plots are normalized so that all experimental bars, and all calculation bars, sum to one, respectively. Full size image The profound difference between atomic carbon and C 60 molecules under intense X-ray exposure is shown by comparing modelled ion yields for atomic carbon with modelled carbon ion yields from C 60 ( Fig. 3 ). For this modelling, the pulse duration was 30 fs and the pulse energy was 345 μJ. The volume-integrated signals were calculated using pulse parameters from the experiment. The huge discrepancy in the C 1+ and C 2+ yields is a direct consequence of atomic Auger (that produces C 2+ from a neutral atom) and molecular Auger effects (that produces two C 1+ ions from neutral atoms in C 60 ), respectively. There is only a small yield of C 3+ ions for the atomic carbon, as the typical ionization channel is the photoionization–Auger emission cycle, which increases the ion charge by 2. This feature of the yields is missing in the fullerene case due to the charge rearrangement assisted by the trapped electron cloud. The relative yield of high charges is more significant for the carbon atom case and suppressed for C 60 because of recombination events. 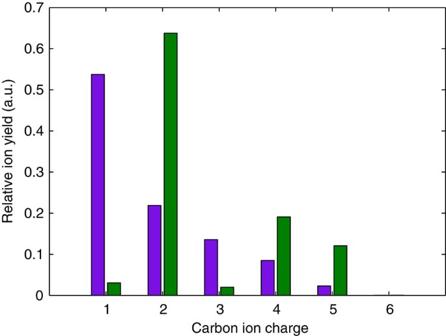Figure 3: Theoretical ion yields for a single carbon atom and C60. For this modelling, the pulse duration was 30 fs and pulse energy was 345 μJ. The green and purple bars stand for single carbon atoms and for C60, respectively. The volume-integrated signals were calculated using pulse parameters from the experiment. The huge discrepancy in the C1+and C2+yields is a direct consequence of atomic Auger (that produces C2+from a neutral atom) and molecular Auger effects (that produces two C1+ions from neutral atoms in C60), respectively. Figure 3: Theoretical ion yields for a single carbon atom and C 60 . For this modelling, the pulse duration was 30 fs and pulse energy was 345 μJ. The green and purple bars stand for single carbon atoms and for C 60 , respectively. The volume-integrated signals were calculated using pulse parameters from the experiment. The huge discrepancy in the C 1+ and C 2+ yields is a direct consequence of atomic Auger (that produces C 2+ from a neutral atom) and molecular Auger effects (that produces two C 1+ ions from neutral atoms in C 60 ), respectively. Full size image For single-carbon atoms at such intense irradiation conditions, the model predicts non-monotonic yields and more abundant highly charged ions than for C 60 , even after volume integration. The different trend of yields indicates charge redistribution in C 60 due to the nanoplasma, while the low yield of highly charged atomic ions in the experiment hints that strong recombination modifies the final charge states after the X-ray pulse ends. Modelling confirms this, as the final average charge state is smaller than the average number of ionization events per atom by up to two charges per atom. Moreover, modelling reveals that the trapped electron evaporation and recombination continues at time scales much longer than the pulse duration. Frustrated absorption and recombination Figure 2 indicates that the yields for high charge states can be reduced by using short pulses. Generally, X-ray photoabsorption is suppressed in high-fluence experiments when the time between successive photoabsorption events is shorter than the Auger lifetimes. This effect has been referred to as frustrated absorption and was observed for atoms [29] and small molecules [34] ; our results show a similar trend for C 60 . 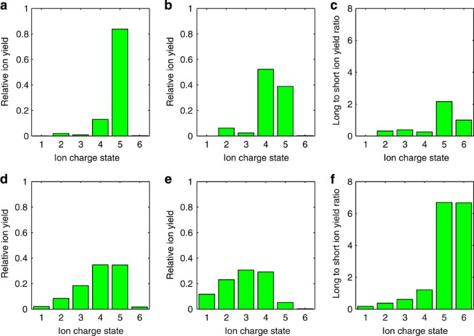Figure 4: Theoretical ion yields for atomic carbon and for C60irradiated for several X-ray pulse durations. For these calculations, a single fluence value (1,400 J cm−2) is considered and volume integration is not performed. (a) Single carbon,T=90 fs; (b) single carbon,T=4 fs; (c) single carbon, ion yield ratios; (d) C60,T=90 fs; (e) C60,T=4 fs; and (f) C60, ion yield ratios. The effect is observable in our modelled data for single-carbon atoms in long (90 fs) and short (4 fs) pulses ( Fig 4a–c ). In Fig. 5a , the suppression of Auger and photoionization events is seen for X-ray fluence over 1,000 J cm −2 . Suppression of high charges is observed for C 60 as well ( Fig. 4d–f ). However, the mechanism is more complex: besides the photoionization and Auger relaxation, secondary ionization and recombination events take part in changing the charge states ( Fig. 5b ). For the short pulse, photoionization is suppressed similarly to the single-atom case. Secondary ionization is most probable for valence electrons, therefore it competes with the Auger process. However, the final average atomic ion charge is much less than the average number of ionizations per atom because of recombination. A stronger attractive potential of the atomic ions can be built up when a shorter pulse is applied that enhances electron trapping, and thus enhances recombination. We conclude that for C 60 , the high charge suppression in the ion yields is due to electron trapping followed by recombination. Figure 4: Theoretical ion yields for atomic carbon and for C 60 irradiated for several X-ray pulse durations. For these calculations, a single fluence value (1,400 J cm −2 ) is considered and volume integration is not performed. ( a ) Single carbon, T =90 fs; ( b ) single carbon, T =4 fs; ( c ) single carbon, ion yield ratios; ( d ) C 60 , T =90 fs; ( e ) C 60 , T =4 fs; and ( f ) C 60 , ion yield ratios. 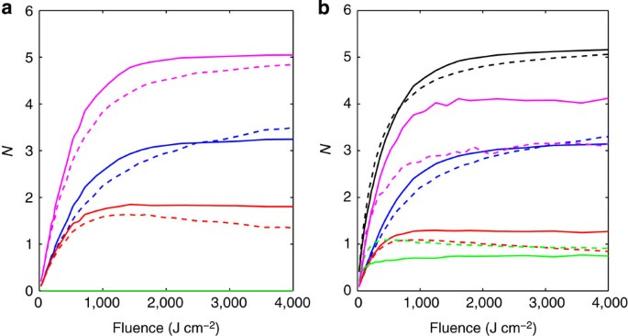Figure 5: Comparison of atomic and molecular absorption versus X-ray pulse peak fluence. Number of ionization events and final charge states per atom for (a) single carbon and (b) C60at long and short pulse durations are shown as a function of fluence. Curves display photoionization events for long (blue solid) and short (blue dashed) pulses, Auger events for long (red solid) and short (red dashed) pulses, secondary ionization events for long (green solid) and short (green dashed) pulses, the sum of all ionization events for long (black) and short (black dashed) pulses and the final charge state after recombination events for long (magenta solid) and short (magenta dashed) pulses. For the single carbon case, there is no secondary ionization, and all ionization events (black) and final charge states (magenta) curves overlap. Full size image Figure 5: Comparison of atomic and molecular absorption versus X-ray pulse peak fluence. Number of ionization events and final charge states per atom for ( a ) single carbon and ( b ) C 60 at long and short pulse durations are shown as a function of fluence. Curves display photoionization events for long (blue solid) and short (blue dashed) pulses, Auger events for long (red solid) and short (red dashed) pulses, secondary ionization events for long (green solid) and short (green dashed) pulses, the sum of all ionization events for long (black) and short (black dashed) pulses and the final charge state after recombination events for long (magenta solid) and short (magenta dashed) pulses. For the single carbon case, there is no secondary ionization, and all ionization events (black) and final charge states (magenta) curves overlap. Full size image Ion KE To understand the temporal evolution of the ionization and Coulomb explosion of C 60 , we examine the dependence of C q + ion KE on the X-ray pulse duration. Measured ion KE distributions show good agreement with the calculations in both mean ion energy and root-mean-squared (RMS) energy spread for short and intermediate pulse durations at near constant X-ray fluence ( Fig. 6 ). The ion KE curves are shown fully in Supplementary Fig. 1 . We observe an almost perfect quadratic scaling of the mean ion KE with ion charge, indicating that the expansion is Coulombic rather than hydrodynamic for C 60 under the X-ray exposure conditions described here ( Supplementary Fig. 2 ). More insight into the Coulomb explosion process is obtained by examining the intra-pulse dynamics using the MD model as shown in Fig. 7 . For highest fluence, the average radius of C 60 starts to grow long before the 90-fs pulse reaches its intensity maximum ( Fig. 7a ) due to the increasing average charge of the atomic ions ( Fig. 7b ). At the peak ( t =0 fs) of the highest fluence X-ray laser pulse, the radius shows a near-linear dependence on time, indicating that the final KEs are approached already on intra-pulse time scales. Thus, the experimental KEs directly reflect the dynamics of the first 100 fs ( Supplementary Fig. 3 ). The average atomic charge state initially increases due to the ionizations, then slowly decreases due to recombination ( Fig. 7b ). At high fluence, the recombination of slow electrons competes with photoionization before the X-ray pulse ends. This process continues for picoseconds as shown in Fig. 7b . 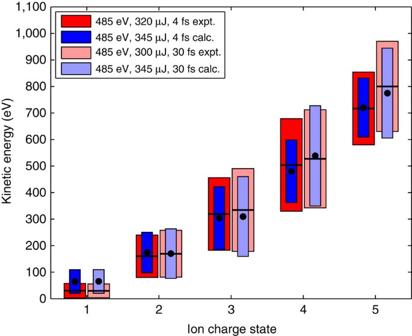Figure 6: Fragment ion KE versus charge state. Experimental data (red/pink rectangles) and calculations (blue/cyan rectangles) are displayed for short and intermediate duration pulses. Mean ion KE versus charge state is indicated by lines (experiment) and circles (simulation) at the centre of each rectangle, while RMS KE width is indicated by the height of each rectangle. Pulse energy in simulation is 345 μJ compared with experimental data taken at 320 μJ (short pulses) and 300 μJ (intermediate pulses). Calc., calculated; expt., experiment. Figure 6: Fragment ion KE versus charge state. Experimental data (red/pink rectangles) and calculations (blue/cyan rectangles) are displayed for short and intermediate duration pulses. Mean ion KE versus charge state is indicated by lines (experiment) and circles (simulation) at the centre of each rectangle, while RMS KE width is indicated by the height of each rectangle. Pulse energy in simulation is 345 μJ compared with experimental data taken at 320 μJ (short pulses) and 300 μJ (intermediate pulses). Calc., calculated; expt., experiment. 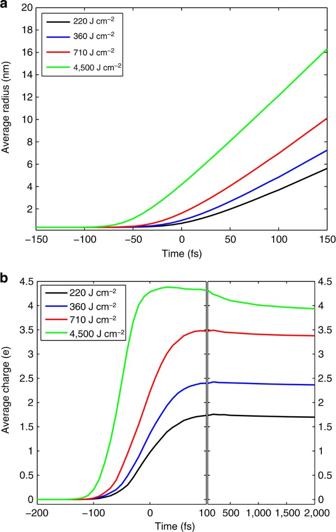Figure 7: Fluence dependence of femtosecond dynamics from simulation. Calculations show average molecule radius (a) and average atomic charge state (b) versus time for long pulses (pulse duration 90 fs) for different fluence values. The molecules expand from an initial average radius of 355 pm. Fluence above 360 J cm−2produces full atomic fragmentation in our calculations. Time zero corresponds to the center of the pulse. Full size image Figure 7: Fluence dependence of femtosecond dynamics from simulation. Calculations show average molecule radius ( a ) and average atomic charge state ( b ) versus time for long pulses (pulse duration 90 fs) for different fluence values. The molecules expand from an initial average radius of 355 pm. Fluence above 360 J cm −2 produces full atomic fragmentation in our calculations. Time zero corresponds to the center of the pulse. Full size image Signatures of molecular effects The impact of the chemical bonds on the mainly Coulomb-driven dynamics is an important question for the simulation of irradiated particles in general. It would seem reasonable to expect that completely neglecting molecular bonds will always result in larger KEs, because we remove attractive binding energy from the system (in the C 60 case it is approximately −430 eV). However, according to our model for the high-fluence intermediate and long pulse cases, neglecting the molecular bonds can in fact have the opposite effect. Without bonds, the ionized part of the system can start to expand very early during the pulse, giving less chance to build up a concentrated high charge and in this way resulting in reduced ion KE ( Fig. 8 ). Notably, this picture is different for the short pulses: atoms within C 60 are ionized so fast that they have no chance to move before bonds are broken. In this regime, bondless modelling yields practically the same KEs and ion yields, indicating that for the high-fluence, short pulse case, the simplification of neglecting chemical bonds in radiation damage calculations is adequate. 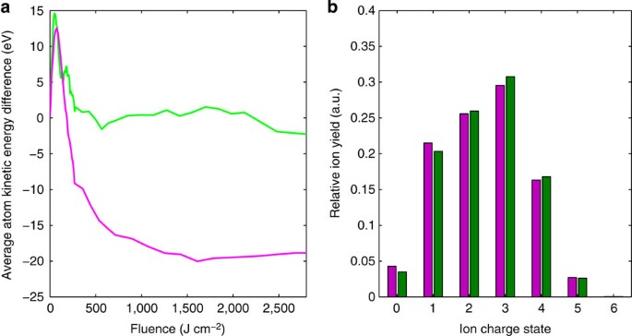Figure 8: Effects of chemical bonds on KEs and ion yields, from simulation. The difference (a) between average atomic KEs obtained from the model without bonds and that obtained from the full model (KEbondless model−KEfull model) are shown for two pulse durations (purple (90 fs), green (4fs)). Atomic ion yields (b) show agreement between the two models (purple for full model and green for full model without bonds) in the short pulse, high-fluence case (in this example, photon energy is 485 eV, pulse duration 4 fs and fluence 550 J cm−2). Under certain conditions, neglect of bonds can be reasonable. For low fluence (fewer ionizations), average atomic KEs are larger for bondless modelling, as expected, but for higher fluence they are smaller. Our modelling indicates that for short (for example, ~5 fs pulse duration), high fluence (above ~500 J cm–2) cases, bondless modelling is adequate. In that regime, there is agreement between the full model and the bondless model for the average atomic KEs (a) and for the atomic ion yields (b). For the short pulse, high fluence case, the difference is almost zero. Figure 8: Effects of chemical bonds on KEs and ion yields, from simulation. The difference ( a ) between average atomic KEs obtained from the model without bonds and that obtained from the full model (KE bondless model −KE full model ) are shown for two pulse durations (purple (90 fs), green (4fs)). Atomic ion yields ( b ) show agreement between the two models (purple for full model and green for full model without bonds) in the short pulse, high-fluence case (in this example, photon energy is 485 eV, pulse duration 4 fs and fluence 550 J cm −2 ). Under certain conditions, neglect of bonds can be reasonable. For low fluence (fewer ionizations), average atomic KEs are larger for bondless modelling, as expected, but for higher fluence they are smaller. Our modelling indicates that for short (for example, ~5 fs pulse duration), high fluence (above ~500 J cm –2 ) cases, bondless modelling is adequate. In that regime, there is agreement between the full model and the bondless model for the average atomic KEs ( a ) and for the atomic ion yields ( b ). For the short pulse, high fluence case, the difference is almost zero. Full size image An XFEL-irradiated molecule such as C 60 displays complex dynamics driven by various physical and chemical phenomena. Modelling enables us to explore the importance of these processes via comparison with experiment. Such general findings can guide the interpretation and theoretical understanding of further high-intensity measurements on complex finite systems. We identify relevant molecular effects by comparing atomic ion yields from different modelling scenarios with the experimental results for two pulse durations (for detailed ion charge state distributions see Supplementary Fig. 4 ) and by quantifying the disagreement between experiment and theory ( Fig. 9 ). We start from a model description where all molecular effects in the 60-atom system are neglected, for example, the carbon atoms can be ionized only by atomic photoionization and intra-atomic Auger effect, but ions and free electrons interact by Coulomb forces and move in real space. The discrepancy is huge: too much C 2+ and too little C 1+ as described earlier, indicating the failure of such simple modelling. To identify the important missing physical and chemical phenomena, a straightforward step is to include bonding by applying force fields. Bonds act against Coulomb repulsion of the ions and allow for molecular fragment formation. As shown in Fig. 9 , the total discrepancy is reduced only slightly because, although C 2+ is somewhat decreased (as atomic ions may be kept in molecular fragments), the relative weight of higher charge states remains strong because the process producing these ions in the high-fluence region is still the same. Drastic improvement reducing the discrepancy by nearly a factor of four is found by switching on secondary ionization: on one hand, the C 1+ production gets stronger (dominantly in lower-fluence regions), while on the other hand trapping of the generated low-energy electrons enhances recombination that suppresses the high charge states from the high-fluence regions. Although the general trend of the yields is captured already (indicated also by the small total discrepancy), further improvement can be achieved by taking into account bond breaking (enhanced C 1+ ion release from molecular fragments) and by introducing molecular Auger effect (enhanced C 1+ ion production against C 2+ ). In conclusion, secondary ionization turns out to be of the highest importance among the molecular phenomena studied even for C 60 , a relatively small molecule when compared with biological macromolecules. This conclusion is also supported by comparison of the KE distributions between modelling and experiment. Therefore, secondary ionization is an essential physical process in all modelling approaches addressing the behaviour of complex systems under high-intensity irradiation. 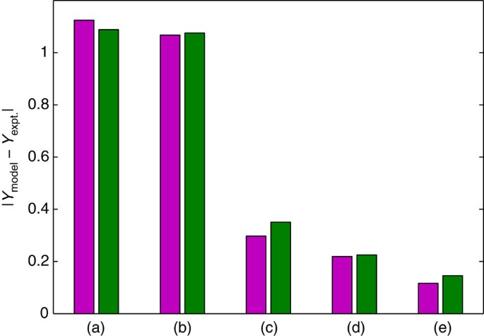Figure 9: Importance of molecular effects in modelling ion yields. Bars display the measure of total discrepancy between ion yields from experiment and from different modelling scenarios (a) without any molecular effects, (b) with bonds added, (c) with bonds and secondary ionization added, (d) with bonds, secondary ionization and bond breaking added, and (e) the full model containing bonds, secondary ionization, bond breaking and the molecular Auger effect (purple bars are for 30 fs while green bars are for 90 fs pulse duration). Atomic ion yields were extracted using a model without any molecular phenomena and other model variants containing an increasing number of effects until reaching the full model (for the ion charge state yields seeSupplementary Fig. 4). For each variant, the absolute differences between experimental and model ion yields were calculated. The sum of the differences over the charge states was then used for a given model to quantify its discrepancy from experiment and was plotted. The comparison clearly shows that all molecular effects are needed for the best agreement, the importance of secondary ionization even for a small molecule as C60, and the failure of a model without any molecular effect. Figure 9: Importance of molecular effects in modelling ion yields. Bars display the measure of total discrepancy between ion yields from experiment and from different modelling scenarios (a) without any molecular effects, (b) with bonds added, (c) with bonds and secondary ionization added, (d) with bonds, secondary ionization and bond breaking added, and (e) the full model containing bonds, secondary ionization, bond breaking and the molecular Auger effect (purple bars are for 30 fs while green bars are for 90 fs pulse duration). Atomic ion yields were extracted using a model without any molecular phenomena and other model variants containing an increasing number of effects until reaching the full model (for the ion charge state yields see Supplementary Fig. 4 ). For each variant, the absolute differences between experimental and model ion yields were calculated. The sum of the differences over the charge states was then used for a given model to quantify its discrepancy from experiment and was plotted. The comparison clearly shows that all molecular effects are needed for the best agreement, the importance of secondary ionization even for a small molecule as C 60 , and the failure of a model without any molecular effect. Full size image Even at high X-ray fluence, the volume-integrated ion fragment mass spectra contain significant quantities of molecular ion fragments (see Supplementary Fig. 5 for molecular fragment ion yields). These larger fragments originate from regions away from the focus where the fluence is not enough to fully destroy all chemical bonds. Modelling correctly predicts the experimentally observed molecular fragment sizes, however, there is larger discrepancy between the yields than in the atomic ion case. The quantitative theoretical description of the larger fragment spectra is a big challenge as chemistry plays a more important role. It is computationally very challenging to carry out quantum simulations to capture the details of bond-breaking mechanisms and fragmentation that happen in parallel with the ionization events. Moreover, even if the computation was feasible, the experimental X-ray laser beam conditions should be better known for a quantitative study. The fragmentation depends strongly on the fluence via the ionization dynamics, therefore the spectra are much more sensitive to the spatiotemporal profile of the XFEL pulse and a more detailed characterization of the X-ray laser beam may be needed than what is available today. This work presents an essential step for the rigorous, quantitative understanding of high-intensity femtosecond X-ray-induced molecular dynamics. Measurements guided the development of MD simulations suitable for large molecules exposed to intense XFEL pulses. Experimental and simulation data on C 60 ion dynamics reveal that a complex variety of physical and chemical processes are present in these interactions. The inclusion of the photoelectric effect, secondary ionization, recombination, as well as molecular Auger processes and chemical bonding in the model produces excellent agreement between experiment and calculation. Our model demonstrates that full atomic fragmentation of C 60 occurs at the highest fluence values. We show that ionization suppression occurs for very short pulses. While an analogous effect is known for atoms and small molecules, the mechanism for such a large molecule is more complex, as revealed by our simulations. Furthermore, our work provides evidence that the charged particles produced by exposing an extended quantum system (C 60 ) to high-fluence X-rays behave as if they were classical particles. Thus, our results present an essential contribution to the validation of a very fundamental assumption underlying all MD modelling approaches, in a previously untested regime. MD modelling is applicable for X-ray interactions with any extended system used in matter in extreme conditions, such as solids, nanosystems and biological macromolecules, even at higher dose rates expected in hard X-ray imaging with future X-ray light sources. Experiment The experiment was conducted at the atomic, molecular and optical physics hutch of the LCLS at SLAC National Accelerator Laboratory using the High Field Physics instrument [17] , [29] , [34] , [46] . X-ray optics focused the incoming X-ray pulses to a peak focal intensity of 10 16 –10 18 W cm −2 . A collimated molecular beam of C 60 molecules from a resistively heated oven crossed the X-ray path at the focus. A magnetic bottle spectrometer, previously used at the LCLS for electron correlation studies [31] , was outfitted with electrostatic lenses, which allowed KE-resolved ion time-of-flight (TOF) spectroscopy with high collection efficiency, even at several hundred eV ion KE. A 2-m-long ion drift path provided high ion mass-to-charge and KE resolution while avoiding overlap of different fragment ion species. The X-ray pulse energy, centroid photon energy and pulse duration were recorded and used as statistical filters in the analysis. The interaction region, defined by the intersection of the focused X-ray beam and the molecular beam, covered a volume around the focus with an inhomogeneous X-ray spatial fluence distribution. Therefore, the measured data contain contributions from a wide range of fluence (volume-integrated signal), with peak X-ray fluence only at the centre of the focus. To model the interaction region, the X-ray spatial fluence distribution was calibrated using ion yields from Ar ( Supplementary Fig. 6 ), which has well-understood sequential multiphoton ionization behaviour [32] . This spatial fluence distribution was then applied in the modelling of the X-ray interaction with C 60 to account for low- and high-fluence regions, allowing quantitative comparison of theoretical predictions with the experimental data. X-ray pulse energies in both experiment and simulation are reported before transmission losses, which average 22% based on the Ar calibration. The X-ray pulse duration was calibrated to the C 60 model based on ion KEs ( Supplementary Fig. 7 ). The calibrated parameters are summarized in Supplementary Table 1 . Magnetic bottle spectrometer outfitted with ion optics To use our magnetic bottle spectrometer, which is frequently used for high detection efficiency electron spectroscopy, as an ion spectrometer, an electrostatic lens system was implemented at the entrance of the 2-m-long flight tube. The permanent magnet located close to the light–matter interaction region was covered with a flat cap to ensure a parallel electrostatic field distribution across the interaction region. Simulations of the spectrometer were carried out using ion trajectory simulation software (SIMION) to determine optimal positions of the lens elements, as well as the corresponding voltages needed for effective ion collection. Ion KE is determined based on ion flight time for each mass-to-charge fragment species according to the spectrometer model. KE-dependent transmission losses are determined by assuming an isotropic ion distribution in the Coulomb explosion. Measured ion KE distributions are modelled in SIMION by least-squares fitting of experimental ion TOF peak shapes with three Gaussian curves, each representing a synthetic KE distribution of the ion with given maximum and width parameters. Where fewer than three curves could produce an adequate fit to the data, fewer curves were used. As an example of the KE analysis method, experimental ion TOF data and least-squares curve fit to the C 3+ peak are shown in Supplementary Fig. 8 . The data were taken with photon energy of 485 eV, pulse energy 900 μJ and pulse duration 90 fs. The ion TOF spectrum exhibits a sharp peak at longer flight times corresponding to low-KE ions, and a broad high-KE peak at shorter flight times originating from the most energetic molecular Coulomb explosions. Pulse-to-pulse statistics from the LCLS diagnostics are used to filter data from the average photon energy and the X-ray pulse energy. For the experimental data presented in this article, pulse energies are < E ›±10% and photon energies are < hν ›±5%. The spectrometer simulations provided the transmission curve versus ion KE for all atomic and molecular fragment ions collected in the experiment. According to the simulations, light ions with low KE are collected with near 100% efficiency, while the transmission declines for more energetic ions within each ion species. Measured atomic ion KE distributions were corrected for the transmission losses based on the spectrometer simulations. For C 2 1+ molecular fragments, spectrometer transmission is nearly 100% for ion KE under 100 eV, then falls to 13% for ion KE above 100 eV. Because the observed ion yield of C 2 1+ approaches zero at KE far less than this 100 eV loss threshold, we estimate 100% collection efficiency for all fragment ions. Care was taken to achieve an overall good collection-detection efficiency instead of optimizing for one specific fragment size or ion KE. Error analysis in ion yields In calculating the ion yields and ion KE, we correct for transmission losses in the spectrometer. SIMION is used to model the transmission versus KE for uniform 4 π spherical initial ion KE distributions, which are split into ‘forward’ (hemisphere directed towards the micro-channel-plates (MCP)) and ‘backward’ (hemisphere initially directed away from MCP) components. The average transmission and TOF distribution of ions with nonzero KE are generally different for the forward and backward components. To fit the measured ion TOF data, we assume equal initial forward and backward ion populations, and find ion KE distributions composed of a sum of three Gaussian curves (in KE) that, when propagated through the simulation, best reproduce the measured ion TOF data. Applying the modelled transmission to the data causes the statistical error of the ion yield measurement to become KE dependent. The directly measured quantity is N i ( t ), the number of ion counts of species i detected at TOF t . Its statistical error (one s.d. of Poisson distribution) is . To estimate the number of ions produced at the focal spot, we need to divide N i ( t ) by the ion collection efficiency, c i ( t ) (this includes both spectrometer transmission and MCP detection efficiency, both dependent on ion KE), which is highest at low KE, and defined by MCP detection efficiency only, but is significantly reduced for ions with high KE due to a larger fraction of ions that miss the detector. Therefore, the relative yield of ions of type i in the focal spot is given by: where R i is the TOF integration range for ions of type i . After integration, the time dependences are removed and we obtain the average collection efficiency c i and total ion counts N i for each ion species i relative to the total average collection efficiency, c tot , for the total number of ions detected, N tot . To find the statistical error on the ion yield, we combine relative statistical errors from N i and N tot : Modelling We applied our atomistic, mixed MD Monte Carlo tool XMDYN [47] , based on a previously developed framework [20] . In this approach, C 60 is treated as 60 individual carbon atoms. Their electronic configuration (for example, the occupancy of the orbitals) is tracked and changed stochastically during every timestep using a Monte Carlo scheme. Cross-sections and rates of the ionization processes calculated by quantum mechanics (XATOM toolkit [48] , [49] ) determine the corresponding probabilities. During ionization events, new classical electrons ‘appear’ in the system with the appropriate energies, as they are released from their bound atomic orbitals. The real-space dynamics of atoms, ions and these (quasi-) free electrons is described by Newtonian mechanics. We applied a multi-timestep position Verlet algorithm with 50 and 0.8 attosecond steps to make modelling on the picoseconds/nanosecond time scales feasible. The atoms are originally held together by a fullerene-specific classical Brenner force field [50] , and charges interact via Coulomb forces. The model contains several physical and chemical processes that were motivated or influenced by the experiment: a molecular Auger effect, secondary ionizations (free electrons colliding with and ionizing atoms/ions) and bond breaking between charged ions. The molecular Auger effect was taken into account by removing the ejected electron from the L shell of a neighbouring atom (if that existed) while the K vacancy of an ion in core-hole state was filled up with its own L electron. Bond breaking due to changes in electronic configuration was modelled by setting the bonding force field to zero between two atomic (charged) ions; the bonding force field was kept if either atom involved was neutral. Recombination of a classically trapped electron occurred within the model if it was no longer delocalized among several ions, but localized to only one ion (recombination to Rydberg states). At the end of the calculation (2 ps after the pulse), some electrons were still trapped but delocalized, which either escaped (by slow evaporation) or recombined at longer times. The number of these escaped electrons was estimated by extrapolation to long times based on the analysis of several sets of trajectories followed up to 0.5 ns. The others were counted to be recombined with the closest ions. Volume-integrated spectra were calculated based on spectra for ~100 different fluence values, calculating 80 realizations for each fixed fluence to improve statistics. A double Gaussian beam profile (a narrower intense hot spot on a wider background) was used in the volume integrations. How to cite this article: Murphy, B. F. et al. Femtosecond X-ray induced explosion of C 60 at extreme intensity. Nat. Commun. 5:4281 doi: 10.1038/ncomms5281 (2014).